2D transition metal dichalcogenides with glucan multivalency for antibody-free pathogen recognition The ability to control the dimensions and properties of nanomaterials is fundamental to the creation of new functions and improvement of their performances in the applications of interest. Herein, we report a strategy based on glucan multivalent interactions for the simultaneous exfoliation and functionalization of two-dimensional transition metal dichalcogenides (TMDs) in an aqueous solution. The multivalent hydrogen bonding of dextran with bulk TMDs (WS 2 , WSe 2 , and MoSe 2 ) in liquid exfoliation effectively produces TMD monolayers with binding multivalency for pathogenic bacteria. Density functional theory simulation reveals that the multivalent hydrogen bonding between dextran and TMD monolayers is very strong and thermodynamically favored (Δ E b = −0.52 eV). The resulting dextran/TMD hybrids (dex-TMDs) exhibit a stronger affinity ( K d = 11 nM) to Escherichia coli O157:H7 ( E. coli ) than E. coli -specific antibodies and aptamers. The dex-TMDs can effectively detect a single copy of E. coli based on their Raman signal. Two-dimensional (2D) transition metal dichalcogenides (TMDs) [1] , [2] , [3] have emerged as a new class of nanomaterials owing to their unique physicochemical properties and potential applications in a variety of research fields including catalysis [4] , [5] , [6] , optoelectronics [7] , biosensing [8] , and energy storage and conversion [9] . In order to fully utilize the outstanding properties of TMDs in the application of interest, monolayered or thin-layered TMD nanosheets are desirable as they exhibit layer-number-dependent electronic structures [10] , [11] . Hence, numerous efforts have been made to develop methods for obtaining thin-layered TMD nanosheets such as mechanical exfoliation [12] , [13] , chemical vapor deposition [14] , [15] , and liquid exfoliation [16] . Among them, liquid exfoliation has many advantages in terms of high production yield, mild condition, and low cost [16] , [17] . Most of the effective liquid exfoliation methods, however, require organic solvents with surface energies close to those of TMD nanosheets. For biological, medical, and sensing applications and aqueous-phase catalysis, however, effective aqua exfoliation of TMD nanosheets without deformation of their electronic structures [18] is essential. To date, several approaches using surfactants [19] , [20] , polymers [21] , [22] , [23] , DNA [24] , and a protein [25] have been developed, but it is still challenging to effectively exfoliate bulk TMDs into TMD monolayers in aqueous solutions and maintain them in a stably dispersed state without aggregation during reactions or assays. In particular, it remains more challenging to impart a specific function to TMD monolayers at the same time as their exfoliation and dispersion during an exfoliation process. The simultaneous exfoliation and functionalization strategy would help reduce efforts required for further modification of TMD nanosheets and improve their performance in the applications of interest. In order to control the simultaneous exfoliation and functionalization of TMD nanosheets in aqueous solutions, it is necessary to investigate and understand the thermodynamic properties of the interactions between TMD nanosheets and exfoliating molecules. The insight into the interactions at the TMD interfaces would enable us to effectively design TMD nanosheets with a specific function, which could be extended to the preparation of a variety of functional 2D nanomaterials. However, the precise understanding of the interactions between the TMD nanosheets and exfoliating molecules in aqueous solutions has been overlooked in most of the previous studies. Pathogenic microorganisms are considered one of the most dangerous elements causing food-borne, water-borne, and air-borne diseases [26] , [27] . Many bacterial pathogens exhibit very low infectious concentrations, which is as low as ten cells for Escherichia coli O157:H7 ( E. coli O157:H7) and Salmonella [28] . One of the most important events occurring during bacterial adhesion and infection is multivalent carbohydrate–lectin interaction [29] , [30] . Hence, it is essential to control these multivalent interactions for devising the strategies for bacteria detection and prevention of infection. Furthermore, the multivalent carbohydrate interactions can be employed for the simultaneous exfoliation and functionalization of TMD nanosheets in aqueous solutions and for bacteria detection. The most widely applied method for bacteria detection is cultivation-based counting, which is, however, very time-consuming and exhibits low sensitivity [31] , [32] . For more sensitive and faster detection of bacteria, polymerase chain reaction (PCR) [33] , [34] and antibody-based immunoassays [35] , [36] have been suggested. PCR-based methods also require multiple sample preparation steps and professional skills, although they are sensitive in bacteria detection [37] . Antibody-based immunoassays exhibit better accessibility to point-of-detection for bacteria as compared to PCR; however, antibodies are expensive and susceptible to perturbation in environmental conditions and they have variable affinities to target antigens, which leads to a diminution in the reproducibility and sensitivity of the assay [28] . Therefore, there is still an increasing demand for a sensing method that achieves the sensitive, selective, rapid, and simple detection of pathogenic bacteria without the use of antibodies [38] . Herein, we report an effective strategy for the simultaneous exfoliation and functionalization of TMD nanosheets in an aqueous solution via multivalent hydrogen bonding of a carbohydrate polymer dextran for the sensitive optical detection of bacteria without the use of antibodies. The thermodynamic binding energy of the multivalent interaction between TMD nanosheets and dextran is also investigated using density functional theory (DFT) calculation. The as-prepared TMD nanosheets with glucan multivalency exhibit a specific recognition capability for E. coli , and are subsequently employed as an optical biosensor for the simple, rapid, and sensitive detection of bacteria in a single copy. Preparation of TMD nanosheets with glucan multivalency Thin TMD nanosheets (WS 2 , WSe 2 , and MoSe 2 ) were exfoliated from bulk TMDs and simultaneously functionalized using a carbohydrate polymer dextran MW 40,000 (denoted “dex”) in an aqueous solution via a simple pulsed sonication process (Fig. 1a ), resulting in dextran/TMD hybrids (denoted as “dex-TMDs”). As investigated in this work, the multivalent hydrogen bonding between the hydroxyl groups of dextran and the chalcogens (S or Se) of TMDs plays an important role in the aqueous phase exfoliation and functionalization of TMD nanosheets. 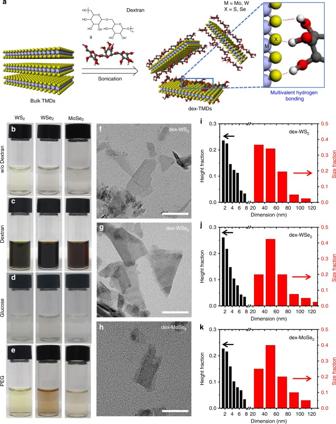Fig. 1 Simultaneous exfoliation and functionalization of TMDs with dextran.aSchematic illustration of the exfoliation and functionalization of TMDs via multivalent hydrogen bonding in an aqueous solution. Photographs of the solution of TMDs exfoliatedbwithout dextran,cwith dextran,dwith glucose, andewith PEG. TEM images offdex-WS2,gdex-WSe2, andhdex-MoSe2(scale bar, 50 nm). Height and lateral size profiles ofidex-WS2,jdex-WSe2, andkdex-MoSe2obtained using AFM Figure 1b shows that none of WS 2 , WSe 2 , and MoSe 2 nanosheets was exfoliated in the absence of dextran in the aqueous solution. However, all the three types of TMD nanosheets were effectively exfoliated in the presence of dextran in the aqueous solution (0.32 mg mL −1 ) as shown in Fig. 1c . In order to demonstrate the importance of multivalent hydrogen bonding in the aqueous phase exfoliation of TMDs, glucose, which is a repeating unit in dextran, was added to a bulk TMD aqueous solution and sonicated under the same condition as dextran. As shown in Fig. 1d , no TMD nanosheets were obtained in the presence of glucose. As the hydrogen bonding multivalency of glucose is two hundred times smaller than that of dextran, the interaction of TMDs with glucose might be too weak to overcome the van der Waals interaction between the TMD interlayers for re-stacking. Furthermore, polyethylene glycol dimethyl ether (PEG, MW 35,000), which cannot undergo hydrogen bonding with TMDs, was added during the exfoliation process (see the Supplementary Methods). As expected, TMD nanosheets were hardly exfoliated in the presence of PEG in the aqueous solution (Fig. 1e ). These results clearly indicate that the multivalent hydrogen bonding of dextran enables the effective exfoliation and functionalization of TMD nanosheets in an aqueous solution. Fig. 1 Simultaneous exfoliation and functionalization of TMDs with dextran. a Schematic illustration of the exfoliation and functionalization of TMDs via multivalent hydrogen bonding in an aqueous solution. Photographs of the solution of TMDs exfoliated b without dextran, c with dextran, d with glucose, and e with PEG. TEM images of f dex-WS 2 , g dex-WSe 2 , and h dex-MoSe 2 (scale bar, 50 nm). Height and lateral size profiles of i dex-WS 2 , j dex-WSe 2 , and k dex-MoSe 2 obtained using AFM Full size image Subsequently, the effect of dextran concentration on the efficiency of exfoliation was investigated. After sonication and centrifugation of the WS 2 solutions containing different amounts of dextran, the absorbance of the obtained solutions at 297 nm was measured to quantify the amount of exfoliated WS 2 nanosheets [22] . When the weight ratio of dextran decreased from 1:3 (bulk TMD:dextran) to 15:1, the exfoliation efficiency of dex-WS 2 nanosheets increased (Supplementary Fig. 1 ). However, as the weight ratio of dextran became less than 15:1, the exfoliation efficiency of dex-WS 2 decreased. The amount of dex-WS 2 nanosheets was additionally quantified by inductively coupled plasma-atomic emission spectroscopy (ICP-AES) (Supplementary Fig. 1c ). The tendency of the exfoliation efficiency measured by ICP-AES over the weight ratios was in good agreement with the UV absorbance-based plot. The highest concentration of dex-WS 2 nanosheets was obtained at a ratio of 15:1. The as-prepared dex-TMD nanosheets were subsequently analyzed using transmission electron microscopy (TEM) and atomic force microscopy (AFM). The TEM images of dex-WS 2 , dex-WSe 2 , and dex-MoSe 2 (Fig. 1f–h ) show that they have a thin layer of 2D nanostructures with an average lateral size of 52 nm (Fig. 1i–k and Supplementary Fig. 2 ). The lattice structures and selected-area electron diffraction (SAED) patterns of dex-TMDs clearly show that they retain an intrinsic 2H phase after exfoliation and functionalization by dextran (Supplementary Fig. 3 ). After removing unbound dextran from the bulk solution via centrifugation, the morphology and thickness of dex-TMDs were measured using AFM. The morphology of dex-WS 2 , dex-WSe 2 , and dex-MoSe 2 appeared rough owing to dextran adsorption on the basal plane of TMDs via multivalent hydrogen bonding (Supplementary Fig. 4 ). Furthermore, the height histograms of dex-TMDs show that the thickness of dex-TMDs was higher than that of monolayer TMDs (Fig. 1i–k ), revealing that 2D TMD nanosheets with multivalent glucan were successfully obtained. Optical properties of dex-TMD nanosheets The optical properties of dex-TMD nanosheets exfoliated in an aqueous solution were investigated. 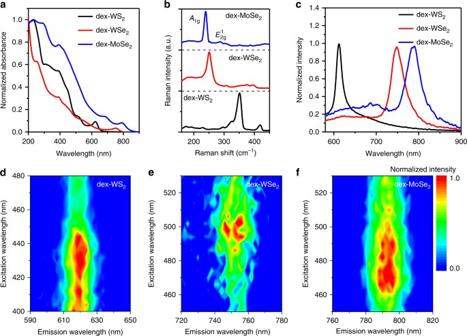Fig. 2 Optical properties of dex-TMDs.aUV–Vis extinction spectra,bRaman spectra, andcphotoluminescence spectra of dex-WS2, dex-WSe2, and dex-MoSe2nanosheets. A 532-nm excitation laser was used. Excitation/emission profiles ofddex-WS2,edex-WSe2, andfdex-MoSe2, demonstrating excitation wavelength-independent photoluminescence Figure 2a shows that the characteristic A excitonic absorption was clearly observed at 621, 752, and 790 nm for dex-WS 2 , dex-WSe 2 , and dex-MoSe 2 , respectively, indicating that all of them maintain semiconducting electronic structures after exfoliation and functionalization [39] . The solution of TMDs exfoliated in the absence of dextran did not produce any characteristic A excitonic absorption peaks (Supplementary Fig. 5 ), indicating that no TMD nanosheets were obtained. To confirm edge and confinement effects on the absorption of dex-WS 2 [20] , [40] , dex-WS 2 was obtained at various centrifugation rates, and then its extinction spectra was taken (Supplementary Fig. 6 ). After normalization of the extinction spectra with the concentration of dex-WS 2 measured by ICP-AES, the extinction coefficient at 235 and 290 nm was plotted as a function of centrifugation rates. The extinction coefficient at 235 nm was independent of the centrifugation rate, whereas the extinction coefficient at 290 nm decreased with increasing the centrifugation rate. It was also found that the wavelength of the A excitonic absorption of dex-WS 2 blue-shifted as the centrifugation rate increased. This result reveals that the edge and confinement effects are valid for dex-WS 2 . Fig. 2 Optical properties of dex-TMDs. a UV–Vis extinction spectra, b Raman spectra, and c photoluminescence spectra of dex-WS 2 , dex-WSe 2 , and dex-MoSe 2 nanosheets. A 532-nm excitation laser was used. Excitation/emission profiles of d dex-WS 2 , e dex-WSe 2 , and f dex-MoSe 2 , demonstrating excitation wavelength-independent photoluminescence Full size image Figure 2b shows the characteristic Raman spectra of dex-WS 2 , dex-WSe 2 , and dex-MoSe 2 . In the Raman spectra of dex-WS 2 (black line), two distinct peaks for a combination of in-plane vibrational mode ( \(E_{2{\mathrm{g}}}^1\) ) and longitudinal acoustic mode (2LA(M)), and an out-of-plane vibrational mode ( A 1g ) appeared at 350 and 418 cm −1 , respectively [41] . As the A 1g mode of WS 2 is more significantly dependent on its layer number than the 2LA(M) mode, their intensity ratio can be used as an indicator to determine the number of WS 2 layers [42] . The intensity ratio of the A 1g peak to the 2LA(M) peak in the Raman spectrum of dex-WS 2 was 6.7, indicating that monolayer dex-WS 2 was mainly exfoliated by dextran. Exfoliated dex-WSe 2 , however, showed only a single Raman signal at 251.7 cm −1 (red line), which is consistent with the result of WSe 2 monolayer reported in other literature [43] . This singlet is considered to be generated by the degeneration of A 1g and E 1 2g modes as the number of WSe 2 decreases to monolayer or a few layers. In the case of MoSe 2 , it is known that the peak position of the A 1g mode depends on the number of MoSe 2 layers, that is, 240 cm −1 for monolayer and the wavenumber increases as the number of layers increases [43] . The A 1g mode of exfoliated dex-MoSe 2 strongly appeared at 239.5 cm −1 (blue line, Fig. 2b ), suggesting that a majority of dex-MoSe 2 nanosheets were monolayers. Subsequently, the photoluminescence (PL) emission of dex-WS 2 , dex-WSe 2 , and dex-MoSe 2 was investigated as shown in Fig. 2c . As compared to bulk WS 2 , strong PL emission of dex-WS 2 appeared at 612 nm (black line, Fig. 2c ), showing the transformation of an indirect semiconductor of bulk WS 2 into a direct semiconductor of WS 2 monolayer. The exfoliated dex-WSe 2 emitted a single PL peak at 748 nm, which distinctly suggests that a majority of WSe 2 nanosheets exfoliated by dextran via multivalent hydrogen bonding were monolayers with a direct band gap (red line). According to previously reported results, two and three layers of WSe 2 exhibited two PL emission peaks at wavelengths longer than 748 nm [20] , [43] . In addition to dex-WS 2 and dex-WSe 2 , dex-MoSe 2 also exhibited characteristic PL emission at 790 nm for monolayers (blue line). In the previous studies, two and three layers of MoSe 2 exhibited their PL emission at wavelengths longer than 800 nm. Subsequently, we measured the excitation and emission profiles of dex-WS 2 , dex-WSe 2 , and dex-MoSe 2 (Fig. 2d–f ). All the dex-TMDs emitted excitation wavelength-independent PL emission with high intensities. Furthermore, it was observed that each dex-TMD had its own excitation wavelength at which its PL emission was the most intense. As reported in the previous literature [20] , we tried to estimate the monolayer volume fraction of dex-WS 2 by applying its PL/Raman intensity ratio to the reported metric. However, the estimated monolayer volume fraction of dex-WS 2 was much lower than what was expected based on its AFM height profile and PL/Raman properties. As discussed in the PL and Raman spectra of dex-WS 2 above, a majority of dex-WS 2 should be monolayers. There are two expected reasons why the previous metric based on a PL/Raman intensity ratio for monolayer volume fractions was not valid for dex-WS 2 . First, the PL intensity of WS 2 nanosheets can be affected by an exfoliating molecule. The quantum yield (QY) of dex-WS 2 might be different from that of surfactant-exfoliated WS 2 nanosheets. Second, the QY of WS 2 nanosheets can be influenced by the extent of defects in which non-radiative recombination takes place, resulting in a decrease in the QY. All the aforementioned optical properties of dex-TMDs demonstrate that bulk TMDs with indirect band gaps were effectively exfoliated into TMD monolayers with direct band gaps via multivalent hydrogen bonding between the hydroxyl groups of dextran and the chalcogens of TMDs in the aqueous solution. Verification of multivalent hydrogen bonding in dex-TMDs We conducted further experiments to verify that the multivalent hydrogen bonding of dextran is a primary factor in the effective exfoliation and functionalization of TMD nanosheets in an aqueous solution. First, a strong hydrogen acceptor, N,N -diisopropylethylamine (DIEA), which can prevent dextran from undergoing multivalent hydrogen bonding with TMDs, was added to the bulk WS 2 solution, followed by sonication. As the concentration of DIEA increased, the color of the exfoliated WS 2 solution collected after centrifugation became lighter and more transparent (Fig. 3a ), indicating that the amount of exfoliated WS 2 nanosheets significantly decreased. Furthermore, the characteristic A1 and B1 excitonic transitions for WS 2 monolayers at 621 and 512 nm significantly decreased in the extinction spectra of the exfoliated solutions obtained in the presence of DIEA, and eventually disappeared as 50 μL of DIEA was added (Fig. 3b and Supplementary Fig. 7 ). This experimental result apparently shows that the multivalent hydrogen bonding of dextran plays a very important role in the exfoliation of TMDs in an aqueous solution. Fig. 3 Multivalent hydrogen bonding in dex-WS 2 nanosheets. a Photographs and b UV–Vis spectra of the solution of WS 2 nanosheets exfoliated and functionalized by dextran in the presence of a proton acceptor DIEA at various concentrations. c FT-IR spectra of dex-WS 2 and dextran, showing hydrogen bonding between WS 2 and dextran. d Absorbance plot of the repeated redispersion of dex-WS 2 after centrifugation, demonstrating that the multivalent hydrogen bonding is sufficiently strong to maintain the stability of the dex-WS 2 colloid in repeated centrifugation-redispersion processes. The absorbance was measured at 621 nm. All error bars represent a standard deviation from the mean values ( n = 4) Full size image Subsequently, we investigated the effect of the chain length of dextran on the exfoliation efficiency of WS 2 . When dextran of MW 1000 (dex1000) was employed in an exfoliation process (Supplementary Fig. 8a ), the color of the obtained solution of exfoliated WS 2 (dex1000-WS 2 ) became lighter and more transparent than the solution of WS 2 nanosheets exfoliated by dextran of MW 40,000 (dex-WS 2 ), indicating that the amount of exfoliated WS 2 nanosheets was reduced as the molecular weight of dextran decreased. Furthermore, two excitonic transitions in the extinction spectrum of dex1000-WS 2 exhibited lower intensity than in the spectrum of dex-WS 2 (Supplementary Fig. 8b ). As discussed, when the chain length was reduced to the extent of a monomer unit (glucose), no TMD nanosheets were exfoliated (Fig. 1d ). These results reveal that the exfoliation efficiency of WS 2 nanosheets decreased as the hydrogen bonding multivalency of dextran was reduced by shortening its chain length. The multivalent hydrogen bonding of dextran with WS 2 nanosheets was directly observed using Fourier transform infrared (FT-IR) spectroscopy. As shown in Fig. 3c , the O–H stretching mode of the hydroxyl groups of dextran in dex-WS 2 was shifted toward a lower frequency (3293 cm −1 ) as compared to that (3349 cm −1 ) of pristine dextran. This peak shift is attributed to the fact that the OH bond strength becomes weak owing to hydrogen bonding with WS 2 . Furthermore, the C–O stretching modes of pristine dextran appeared very broad at approximately 1004 cm −1 owing to intramolecular hydrogen bonding [44] . However, the C–O stretching modes in dex-WS 2 nanosheets appeared sharp and were more clearly resolved at 1046, 1021, and 993 cm −1 , because the dextran on the basal plane of WS 2 mostly underwent intermolecular hydrogen bonding—rather than intramolecular hydrogen bonding—with the sulfur atoms. In the X-ray photoelectron spectroscopy spectra of dex-WS 2 (Supplementary Fig. 9 ), the characteristic peaks of dextran were also observed, demonstrating that dex-WS 2 hybrids were successfully prepared. Moreover, the W 4f peaks of dex-WS 2 confirmed that it retained an intrinsic 2H phase after exfoliation and functionalization. It was observed that dex-WS 2 was partially oxidized to produce tungsten oxide during a process of exfoliation. The tungsten oxide content in dex-WS 2 increased to 31% as compared to the proportion (15%) of starting bulk WS 2 . However, the tungsten oxide content in dex-WS 2 significantly decreased to 21% as the sonication amplitude was reduced to a half. Subsequently, the stability of multivalent hydrogen bonding in dex-WS 2 nanosheets was investigated by measuring their colloidal stability. After removing unbound dextran from the bulk solution, dex-WS 2 underwent a repeated centrifugation and re-dispersion process. The A excitonic absorption at 621 nm was then measured at each stage to determine the colloidal stability of dex-WS 2 (Fig. 3d ). The absorption of dex-WS 2 remained constant even after repeated centrifugation and re-dispersion, indicating that dex-WS 2 maintained the stability of its hybrid structure without aggregation. Furthermore, dex-WS 2 was stably dispersed without re-aggregation for 2 months. These results suggest that multivalent hydrogen bonding in dex-WS 2 is sufficiently strong to maintain the stability of the hybrid nanostructure in an aqueous solution for a certain duration. DFT calculation for the interaction between dextran and TMDs We conducted computational DFT simulation to calculate the thermodynamic properties of the interactions between dextran and TMD nanosheets. First, we calculated the interaction potential energy between two parallel monolayers of WS 2 in the presence or absence of dextran as a function of the interlayer distance. As shown in Fig. 4a, b , the interaction potential energy of the WS 2 interlayer was noticeably lower in the presence of dextran during the exfoliation process in the aqueous solution as compared to the value calculated in the absence of dextran. This reduced potential energy clearly reveals that the exfoliation of TMD nanosheets in the aqueous solution can be facilitated by the incorporation of dextran and they can be stably dispersed with lower tendency toward re-aggregation. Accordingly, the required energy for the exfoliation of WS 2 monolayer in the presence of dextran is significantly reduced from 5 to 1 eV for an increase in the interlayer distance of 2 Å from the most stable distance. Fig. 4 DFT simulation for the interactions between dextran and TMD. Potential energy of interaction between two parallel monolayers of WS 2 a with and b without dextran. The central image illustrates an exfoliation process in two cases. Binding energy of the hydrophilic hydroxyl groups of dextran with c pure WS 2 , d oxygen-defective WS 2 , and e hydroxyl-defective WS 2 Full size image Subsequently, we calculated the binding energy of the hydrophilic hydroxyl groups of dextran on the surface of pure WS 2 or defective WS 2 monolayers. As shown in Fig. 4c , the binding energy of the hydrophilic part of dextran with pure WS 2 not bearing any defects was determined to be −0.24 eV, which is already thermodynamically favored. If a WS 2 nanosheet has an oxygen defect (Fig. 4d ), the binding energy becomes a greater negative value (−0.32 eV), indicating that the interaction between dextran and the WS 2 nanosheet can be stronger. Furthermore, the binding energy of dextran with a hydroxyl-defective WS 2 nanosheet was determined to be a greater negative value (−0.52 eV) than that with an oxygen-defective WS 2 nanosheet (Fig. 4e ). As these defective WS 2 nanosheets can be produced during the exfoliation process (Supplementary Fig. 9 ), three types of interactions between dextran and WS 2 nanosheets are likely to occur in the aqueous solution. The simulation results clearly show that the hydroxyl groups of dextran can forge strong bonds with pure and defective WS 2 monolayers, which is sufficient to exfoliate and stably disperse them without re-aggregation in the aqueous solution. In particular, the exfoliation of TMD monolayers can be further facilitated by the multivalent binding of dextran, which leads to much stronger interactions in the TMD hybrids as observed in carbohydrate–lectin interactions. Antibody-free recognition of pathogenic bacteria E. coli O157:H7 is a Gram-negative pathogen with carbohydrate binding sites such as Type 1 fimbriae ( fim ) and pyelonephritis-associated pili ( pap ) containing the fim H protein [45] , [46] . The fim H lectin is known as a mannose-binding protein ( K d = 2.3 μM), but it also has a very low binding affinity to glucose ( K d = 9.4 mM). The low binding affinity of this lectin to glucose inspires us to design dex-TMD nanosheets with glucan multivalency for improved and antibody-free recognition of E. coli . We hypothesize that dex-TMDs with glucose multivalency would enable selective recognition of E. coli O157:H7 with a significantly enhanced binding affinity against other pathogenic bacteria. In order to confirm our hypothesis, three different types of pathogenic bacteria— E. coli O157:H7, Salmonella typhimurium (Gram-negative), and Staphylococcus ( S .) aureus (Gram-positive)—were incubated with dex-WS 2 in a separate reaction vessel for 1 h (Fig. 5a , see the Supplementary Methods for bacteria culture). After washing each bacteria with phosphate-buffered saline (PBS) to remove unbound dex-WS 2 , the optical photograph of a pile of bacteria centrifuged was taken (Supplementary Fig. 10a ). The dex-WS 2 -treated E. coli turned light yellow from white after reaction with dex-WS 2 , indicating that dex-WS 2 bound on the surface of the bacteria. However, Salmonella typhimurium and S . aureus retained an original white color even after reaction with dex-WS 2 , indicating that dex-WS 2 hardly bound on these bacteria. Then, the dex-WS 2 -treated bacteria (2 × 10 6 colony-forming unit (CFU)) were placed on glass microarrays for detection by measuring the Raman scattering signals (2LA(M), E 1 2g and A 1g ) of dex-WS 2 bound on the bacteria (Fig. 5b, c ). As shown in the results of ensemble measurement (Fig. 5d ), strong Raman signals of dex-WS 2 were observed only from E. coli . Negligible Raman signals were measured from both Salmonella typhimurium and S . aureus as shown in the Raman images generated by the intensity of the 2LA(M) peak of dex-WS 2 . The total intensity of dex-WS 2 obtained from the three types of bacteria demonstrates that dex-WS 2 with glucan multivalency could selectively recognize E. coli against Salmonella typhimurium and S . aureus (Fig. 5e ). The content of dex-WS 2 bound on the bacteria was further quantified using ICP-AES (Supplementary Fig. 10b ). A large amount of WS 2 (6.95 μg mL −1 ) was measured from the dex-WS 2 -treated E. coli , whereas a trace amount of WS 2 was observed from the dex-WS 2 -treated Salmonella typhimurium and S . aureus . This is in good agreement with the result of the bacterial detection based on the Raman signal measurement on glass microarrays. This result reveals again that dex-WS 2 was able to recognize E. coli without the use of antibodies. Fig. 5 Antibody-free optical detection of bacteria with dex-WS 2 . a Schematic illustration of the antibody-free optical detection of bacteria with dex-WS 2 . b Glass microarray and c Optical photographs of E. coli , Salmonella typhimurium , and S. aureus (2×10 6 CFU) treated with dex-WS 2 (25 μg mL −1 ) (scale bar, 500 μm). d Raman images of the dex-WS 2 -treated bacteria based on the 2LA(M) peak of dex-WS 2 at 352 cm −1 , showing the selective recognition of E. coli . e The total intensity of the Raman signal of dex-WS 2 bound on three different types of bacteria. f E. coli detection as a function of dex-WS 2 concentrations for the extraction of its affinity to E. coli . g Langmuir isotherm for the binding of dex-WS 2 to E. coli . All error bars represent a standard deviation from the mean values ( n = 4) Full size image Notably, the Raman signals (2LA(M) and A 1g ) of dex-WS 2 remained very intense with almost the same intensity even after binding on E. coli whereas its fluorescence was completely quenched (Supplementary Fig. 11 ). This fluorescence quenching of dex-WS 2 might be caused by the energy transfer to a variety of proteins on E. coli or the charge transfer to K + ions released out of the bacteria as previously observed in quasi-2D MoS 2 adsorbed on yeast cells [47] . To investigate further the selectivity of dex-WS 2 to E. coli O157:H7, other strains of E. coli such as E. coli K-12 and E. coli O1:K1:H7 were incubated with dex-WS 2 , and then the 2LA(M) Raman signals at 352 cm −1 were collected from the bacteria on glass microarrays. As shown in Fig. 6 , the strong Raman signals of dex-WS 2 were observed only from E. coli O157:H7. The very weak Raman signals of dex-WS 2 were measured from both E. coli K-12 and E. coli O1:K1:H7. This result clearly reveals that dex-WS 2 was able to effectively recognize E. coli O157:H7 against other strains of E. coli . It is worth noting that dex-WS 2 could differentiate E. coli O157:H7 from other strains of E. coli K-12 and E. coli O1:K1:H7, although they all have fim H on their membrane [48] , [49] . We speculate that the increased binding affinity of dex-WS 2 to E. coli O157:H7 might be ascribed to the fact for the slight structural difference of the fim H on the E. coli or the recognition capability of a three-dimensional structure of dextran created on the rigid surface of WS 2 nanosheets. Fig. 6 Recognition selectivity of dex-WS 2 to different strains of E. coli . a Raman images of the dex-WS 2 -treated bacteria based on the 2LA(M) peak of dex-WS 2 at 352 cm −1 , showing the effective recognition of E. coli O157:H7 against E. coli K-12 and E. coli O1:K1:H7. b The normalized total intensity of the 2LA(M) Raman signal of dex-WS 2 bound on three different strains of E. coli . All error bars represent a standard deviation from the mean values ( n = 4) Full size image We calculated the binding affinity of dex-WS 2 to E. coli . As shown in Fig. 5f , the Raman signal of dex-WS 2 from E. coli gradually increased when its concentration increased in the reaction with the bacteria, indicating that the binding kinetics of dex-WS 2 exhibit a concentration dependency. This concentration-dependent response was subsequently fitted with the Langmuir isotherm to extract the dissociation constant ( K d ) of dex-WS 2 for binding with E. coli (Fig. 5g , see the details in the Supplementary Methods). The obtained K d value was 11 nM, which is much lower than the reported values for a monoclonal antibody, an aptamer specific for the bacteria [50] , [51] , and mannose. This lower K d value suggests that dex-WS 2 with glucan multivalency has a higher binding affinity to E. coli than the antibody, aptamer, and mannose, which leads to the sensitive recognition of the target bacteria. We additionally measured the binding affinity of dex-WS 2 and an E. coli -specific antibody using a quartz crystal microbalance (QCM), and compared their binding affinity to E. coli O157:H7 (Supplementary Fig. 12 , see the details in the Supplementary Methods). The QCM measurement reveals again that dex-WS 2 exhibited a higher binding affinity to E. coli O157:H7 than the E. coli -specific antibody. This significantly enhanced binding affinity of dex-WS 2 can be attributed to its multivalent binding ability for lectins on E. coli . Subsequently, a single copy of bacteria was detected with dex-WS 2 (see the Supplementary Methods). After the reaction of E. coli , Salmonella typhimurium , or S. aureus with dex-WS 2 , very dilute bacteria solution was spotted on microarrays for the Raman imaging based on its 2LA(M) peak at 352 cm −1 . As shown in Fig. 7 , a very intense Raman signal of dex-WS 2 was observed from the single copy of E. coli whereas there was no noticeable Raman signal from both Salmonella typhimurium and S . aureus . Furthermore, when the dex-WS 2 -treated E. coli was analyzed using scanning electron microscopy, dex-WS 2 nanosheets were clearly observed on the surface of the treated E. coli , whereas no nanosheets were observed on pristine E. coli (Supplementary Fig. 13 ). These results reveal that dex-WS 2 nanosheets with glucan multivalency were able to effectively detect E. coli pathogens in a single copy without the use of antibodies. Fig. 7 Detection of a single copy of bacteria with dex-WS 2 . a Optical photographs of distinctly spread single bacterium. b Raman mapping of the single bacterium treated with dex-WS 2 based on the Raman scattering peak at 352 cm −1 , demonstrating that dex-WS 2 nanosheets could selectively detect E. coli at single copy level (scale bar, 2 μm) Full size image As compared to previous methods for bacteria detection, this sensing method based on dex-TMDs with glucan multivalency has many advantages: the sensing material dex-TMDs can be more readily prepared and are not significantly susceptible to perturbation in physical conditions. Furthermore, the dex-TMD sensing method enables the fast, simple, sensitive, and cost-effective detection of pathogenic bacteria. Glucan multivalent interactions facilitated the simultaneous exfoliation and functionalization of TMD nanosheets in an aqueous solution, resulting in dex-TMD hybrids with a specific function for the selective recognition of E. coli without the use of antibodies. Experimental data and DFT simulation revealed that multivalent hydrogen bonding of dextran was a primary factor in the effective exfoliation and stable functionalization of TMD nanosheets in the aqueous solution. Furthermore, the multivalent hydrogen bonding of dextran with TMD nanosheets was observed to be very strong and thermodynamically favored. The as-prepared dex-TMDs were able to selectively detect a single copy of E. coli without the use of antibodies. 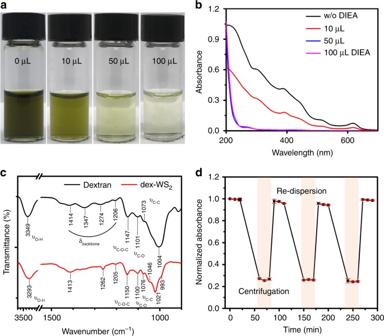Fig. 3 Multivalent hydrogen bonding in dex-WS2nanosheets.aPhotographs andbUV–Vis spectra of the solution of WS2nanosheets exfoliated and functionalized by dextran in the presence of a proton acceptor DIEA at various concentrations.cFT-IR spectra of dex-WS2and dextran, showing hydrogen bonding between WS2and dextran.dAbsorbance plot of the repeated redispersion of dex-WS2after centrifugation, demonstrating that the multivalent hydrogen bonding is sufficiently strong to maintain the stability of the dex-WS2colloid in repeated centrifugation-redispersion processes. The absorbance was measured at 621 nm. All error bars represent a standard deviation from the mean values (n= 4) In addition, the dex-TMDs could differentiate E. coli O157:H7 from other strains of E. coli such as E. coli K-12 and E. coli O1:K1:H7. This exfoliation and functionalization approach based on multivalent hydrogen bonding can be extended to other 2D nanomaterials to design diverse hybrids with new functions. Moreover, the antibody-free sensing method based on dex-TMDs with binding multivalency can evolve into nanosensors capable of both detection and therapy of various diseases. Synthesis of TMD nanosheets with glucan multivalency In this study, dex-TMD nanosheets were obtained via liquid exfoliation of bulk TMDs in the presence of dextran (MW 40,000) in water. Accordingly, 6 g of bulk TMD (8.4 g for WSe 2 ) was added to 200 mL of water containing dextran (2 g L −1 ), followed by sonication using a tip sonicator in an ice bath for 5 h at 75% amplitude with a pulse of 6 s on and 2 s off. 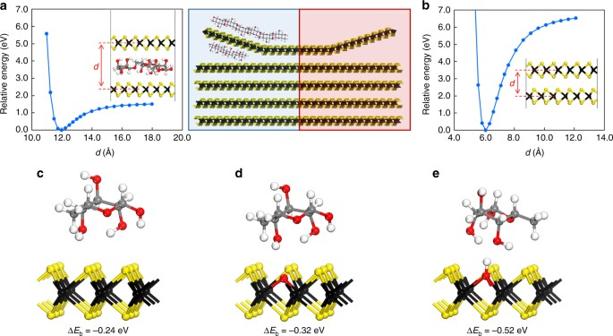Fig. 4 DFT simulation for the interactions between dextran and TMD. Potential energy of interaction between two parallel monolayers of WS2awith andbwithout dextran. The central image illustrates an exfoliation process in two cases. Binding energy of the hydrophilic hydroxyl groups of dextran withcpure WS2,doxygen-defective WS2, andehydroxyl-defective WS2 The resulting solution was centrifuged at 1977 × g for 1.5 h to discard unexfoliated TMDs. The supernatant was collected and centrifuged again at 15,344 × g for 1.5 h. The sediment was collected, but the supernatant was discarded to remove unbound dextran and a smaller size of TMD particles. Subsequently, the sediment obtained at 15,344 × g was re-dispersed in 25 mL of water and centrifuged again at 3024 × g for 1.5 h. The supernatant solution was finally collected to obtain dex-TMD monolayers (3024–15,344 × g ). DFT calculation for the interaction between dextran and TMDs All ab initio calculations were performed with the Vienna Ab initio Simulation Package (VASP 5.4.1) [52] , [53] , [54] , [55] using the projector augmented wave method [56] , [57] with the generalized gradient approximation based on the Perdew–Burke–Ernzerhof exchange-correlation functional [58] , [59] . In order to consider van der Waals interaction, the DFT + D3 method [59] , in which the dispersion coefficients depend on the local structural geometry, was included in this work. Periodic boundary conditions were used in all directions and 20 Å of vacuum was used in the z -direction to separate the slabs. A plane-wave cutoff energy of 500 eV was employed to control the fineness of this mesh. All the calculations were carried out using fully optimized structures, where lattice vectors and ionic positions were fully relaxed until the maximum atomic forces were <0.04 eV Å −1 . General procedure for the detection of bacteria with dex-TMDs First, 100 μL of dex-TMD (125 μg mL −1 ) was dispersed in 500 μL of PBS (10 mM, pH 7.4). Subsequently, 50 μL of bacteria was added to the dex-TMD solution, in which the final concentration of bacteria was 10 8 CFU mL − 1 . The resulting mixture was incubated for 1 h at 25 °C (500 rpm, Thermomixer). 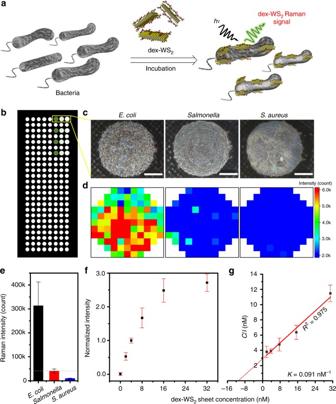Fig. 5 Antibody-free optical detection of bacteria with dex-WS2.aSchematic illustration of the antibody-free optical detection of bacteria with dex-WS2.bGlass microarray andcOptical photographs ofE. coli,Salmonella typhimurium, andS. aureus(2×106CFU) treated with dex-WS2(25 μg mL−1) (scale bar, 500 μm).dRaman images of the dex-WS2-treated bacteria based on the 2LA(M) peak of dex-WS2at 352 cm−1, showing the selective recognition ofE. coli.eThe total intensity of the Raman signal of dex-WS2bound on three different types of bacteria.fE. colidetection as a function of dex-WS2concentrations for the extraction of its affinity toE. coli.gLangmuir isotherm for the binding of dex-WS2toE. coli. All error bars represent a standard deviation from the mean values (n= 4) The reaction mixture was centrifuged for 5 min (4 °C, 1977 × g ) to collect the bacteria and remove unbound dex-TMDs. The collected bacteria were thereafter washed with PBS several times to further remove unbound dex-TMDs in the solution. 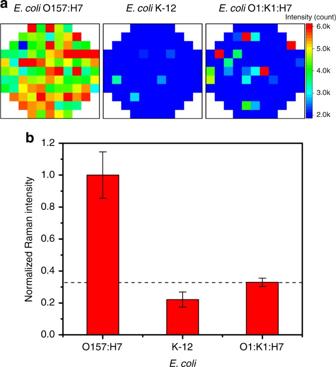Fig. 6 Recognition selectivity of dex-WS2to different strains ofE. coli.aRaman images of the dex-WS2-treated bacteria based on the 2LA(M) peak of dex-WS2at 352 cm−1, showing the effective recognition ofE. coliO157:H7 againstE. coliK-12 andE. coliO1:K1:H7.bThe normalized total intensity of the 2LA(M) Raman signal of dex-WS2bound on three different strains ofE. coli. All error bars represent a standard deviation from the mean values (n= 4) 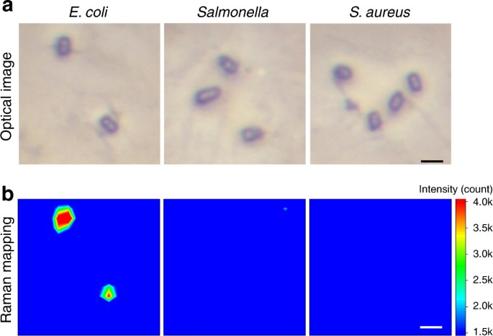Fig. 7 Detection of a single copy of bacteria with dex-WS2.aOptical photographs of distinctly spread single bacterium.bRaman mapping of the single bacterium treated with dex-WS2based on the Raman scattering peak at 352 cm−1, demonstrating that dex-WS2nanosheets could selectively detectE. coliat single copy level (scale bar, 2 μm) After the addition of 50 μL of PBS to the bacteria sediment, 2 μL of the bacteria solution (2×10 6 CFU) was placed on glass microarrays for measurement. Data availability All the data supporting the findings of this work are available on the article and its Supplementary Information files and/or from the corresponding author upon request.